Carbon dioxide concentration dictates alternative methanogenic pathways in oil reservoirs Deep subsurface formations (for example, high-temperature oil reservoirs) are candidate sites for carbon capture and storage technology. However, very little is known about how the subsurface microbial community would respond to an increase in CO 2 pressure resulting from carbon capture and storage. Here we construct microcosms mimicking reservoir conditions (55 °C, 5 MPa) using high-temperature oil reservoir samples. Methanogenesis occurs under both high and low CO 2 conditions in the microcosms. However, the increase in CO 2 pressure accelerates the rate of methanogenesis to more than twice than that under low CO 2 conditions. Isotope tracer and molecular analyses show that high CO 2 conditions invoke acetoclastic methanogenesis in place of syntrophic acetate oxidation coupled with hydrogenotrophic methanogenesis that typically occurs in this environment (low CO 2 conditions). Our results present a possibility of carbon capture and storage for enhanced microbial energy production in deep subsurface environments that can mitigate global warming and energy depletion. Carbon capture and storage (CCS) is a candidate technology to reduce the emission of CO 2 from factories and power plants [1] , [2] . The underlying idea is to capture CO 2 rather than emitting it into the atmosphere and to sequester it in deep subsurface formations such as deep saline aquifers or depleted oil and gas reservoirs [3] . This technology has the potential to reduce future global CO 2 emissions by 20% [2] , [4] . The economical and technological feasibilities of CCS have been extensively studied over the past decade, mainly from a geological perspective [5] , [6] , [7] , [8] . Recently, microbial effects associated with CO 2 storage also have been investigated in deep saline aquifers [9] , [10] , and the influence of CO 2 injection on microbial community structure has been reported. A study revealed that CO 2 injection changed the constituent of methanogens and sulfate reducers in the deep subsurface microbial community [10] . Oil reservoirs are also unique subsurface environments that are potential repositories for CO 2 sequestration [11] , [12] and often harbor active methane-producing microbial communities [13] , [14] , [15] . However, very little is known about the effect of CO 2 sequestration on microbial communities and their functional role in deep subsurface oil reservoirs. In the present study, we aimed to reveal how the microbial community and functions associated with methanogenesis respond to the increase in CO 2 concentration in the oil reservoirs. We performed laboratory experiments that simulated field conditions from where samples were collected. Based on stable isotope tracer analysis, molecular analysis and thermodynamic calculations, we report the possibility that drastic changes of microbial communities and methanogenic functions can be induced by CO 2 injection into deep subsurface high-temperature oil reservoirs. Effect of CO 2 on methanogenesis in oil field microcosms We selected a high-temperature oil reservoir, Yabase oil field, Japan, where we previously demonstrated the occurrence of in situ methanogenic activity [15] . Acetate, which is highly abundant in this reservoir (6–9 mM), is a primary precursor to methane. We previously found that methane was produced from acetate via syntrophic acetate oxidation coupled with hydrogenotrophic methanogenesis in the reservoir [15] . To determine if methanogenesis would continue if CO 2 concentrations increased in subsurface oil reservoirs, we set up high-temperature and high-pressure incubation apparatuses (working volume: 1 l; Supplementary Fig. S1 ), mimicking the in situ oil reservoir (1,000–1,300 m deep, 53–65 °C, 5 MPa; Supplementary Table S1 ). Production water from the reservoir used in this study contained 6.4 mM of acetate, 39.6 mM of bicarbonate and indigenous microbes. We inoculated 8 ml of crude oil and 800 ml of the production water as a source of indigenous microbes and nutrients into the apparatuses, pressurized with either N 2 or N 2 /CO 2 (90:10) gas to a final pressure of 5 MPa, and incubated at 55 °C. The microcosms incubated under an N 2 atmosphere were designated ‘control microcosms’, and those incubated under an N 2 /CO 2 atmosphere were designated as ‘CO 2 -injected microcosms’. Control and CO 2 -injected microcosm experiments were prepared in triplicate. Two of the three microcosms were amended with either a trace amount of 13 C-bicarbonate (final 400 μM) or [2- 13 C]-acetate (final 87.5 μM) to track the methanogenic pathway. After 1 week of incubation, CO 2 partial pressures and bicarbonate concentrations in the control microcosms stabilized at ~0.004 MPa (=0.04 atm) and 47.7 mM and in the CO 2 -injected microcosms at 0.2 MPa (=2.0 atm) and 86.4 mM; decrease in CO 2 was due to dissolution into the production water. The pH levels in both microcosms were stable at ~8.2 and 7.3, respectively, during incubation. The conditions in the CO 2 -injected microcosms were likely to reflect the bicarbonate concentration and pH in previously reported CCS sites ( Supplementary Table S1 ). In all microcosms, methane productions increased after at least 50 days of incubation, whereas methane productions in CO 2 -injected microcosms completed ~30 days earlier than the control microcosms ( Fig. 1a ). Acetate present in the original production water decreased concomitantly with increased methane production. Methane production and acetate degradation in microcosms labeled with stable isotope tracers were almost similar to unlabeled microcosms. Methane production was nearly equivalent to the acetate consumed. This stoichiometric methanogenic reaction suggests that almost all the methane formed was derived from acetate. Interestingly, the methane production rate in CO 2 -injected microcosms (0.36±0.04 μmol d −1 ml −1 water at the growing phase) was twice as high as in control microcosms (0.17±0.02 μmol d −1 ml water at the growing phase), indicating that CO 2 injection stimulated methanogenesis. 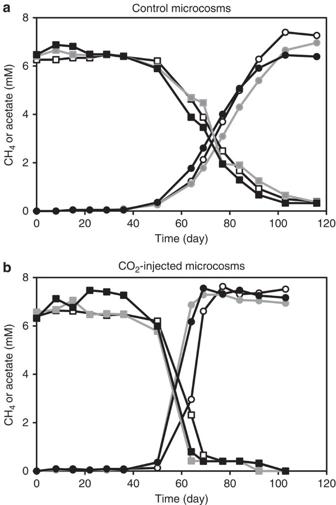Figure 1: Methanogenesis in control and CO2-injected microcosms. Methanogenesis shown in (a) three individual control microcosms and (b) three individual CO2-injected microcosms under high-temperature and high-pressure conditions (55 °C and 5 MPa). Methane (circles) and acetate (squares) concentrations over time in the unlabeled (closed symbols), [2-13C]-acetate (gray symbols) and13C-bicarbonate (open symbols)-labeled microcosms. All six microcosms were constructed using high-temperature oil reservoir samples. Figure 1: Methanogenesis in control and CO 2 -injected microcosms. Methanogenesis shown in ( a ) three individual control microcosms and ( b ) three individual CO 2 -injected microcosms under high-temperature and high-pressure conditions (55 °C and 5 MPa). Methane (circles) and acetate (squares) concentrations over time in the unlabeled (closed symbols), [2- 13 C]-acetate (gray symbols) and 13 C-bicarbonate (open symbols)-labeled microcosms. All six microcosms were constructed using high-temperature oil reservoir samples. Full size image CO 2 -driven change in methanogenic pathway in microcosms To identify the methanogenic pathways in the control and CO 2 -injected microcosms, the carbon isotopic compositions (δ 13 C) of methane and dissolved inorganic carbon (DIC) were measured during incubation. In the control microcosms labeled with 13 C-bicarbonate, elevated δ 13 C methane values (>450‰) were detected ( Fig. 2a ), showing that the amended 13 C-bicarbonate was converted to 13 CH 4 . In the [2- 13 C]-acetate-labeled control microcosm, δ 13 C DIC values gradually increased and methane also became enriched in 13 C following DIC ( Supplementary Table S2 ), indicating that the 13 C-methyl group of acetate was oxidized to CO 2 and incorporated into a large CO 2 pool, and a small fraction of 13 CO 2 was converted to 13 CH 4 (acetate oxidation: CH 3 COO − +H + +2H 2 O→4H 2 +2CO 2 ; methanogenesis from H 2 : 4H 2 +CO 2 →CH 4 +2H 2 O; over all, CH 3 COO − +H + →CH 4 +CO 2 ). In contrast, the [2- 13 C]-acetate added to a CO 2 -injected microcosm resulted in elevated δ 13 C methane values (>850‰) ( Fig. 2b ). This indicates that the 13 C-methyl group of acetate was directly converted to 13 CH 4 ( 13 CH 3 COO − +H + → 13 CH 4 +CO 2 ). These observations demonstrated that the dominant methanogenic pathway in the control microcosms was syntrophic acetate oxidation coupled with hydrogenotrophic methanogenesis, while acetoclastic methanogenesis was the dominant methanogenic pathway in the CO 2 -injected microcosms. The values of carbon isotopic fractionation between CH 4 and DIC in the unlabeled control ( ε C =−83.3±1.3‰) and CO 2 -injected ( ε C =−10.9±1.0‰) microcosms during incubation ( Supplementary Table S2 ) were also consistent with the hydrogenotrophic and acetoclastic methanogenesis, respectively [16] . The reproducibility of the impact of CO 2 on the methanogenic pathway and community resiliency were confirmed by an additional stable isotope tracer experiment, which showed that the dominant methanogenic community and pathway switched from one to the other when the headspace gas of the control microcosm was replaced with N 2 /CO 2 (90:10) and the CO 2 -injected microcosm was replaced with 100% N 2 ( Supplementary Note 1 ; Supplementary Figs. S2 and S3 , and Supplementary Tables S3, S4 and S5 ). 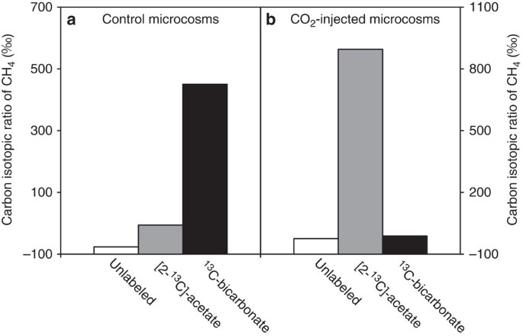Figure 2: Carbon isotopic ratios of methane in control and CO2-injected microcosms after incubation. Carbon isotopic ratios of methane in the (a) control microcosms and (b) CO2-injected microcosms after incubation of 103 days. Carbon isotopic ratios of methane and dissolved inorganic carbon (DIC) in each microcosm during incubation are shown inSupplementary Table S2. Figure 2: Carbon isotopic ratios of methane in control and CO 2 -injected microcosms after incubation. Carbon isotopic ratios of methane in the ( a ) control microcosms and ( b ) CO 2 -injected microcosms after incubation of 103 days. Carbon isotopic ratios of methane and dissolved inorganic carbon (DIC) in each microcosm during incubation are shown in Supplementary Table S2 . Full size image CO 2 -induced alteration of methanogenic microbial community Quantitative PCR (qPCR) and 16S rRNA gene clone library analysis showed differences in microbial community structure in the original production water compared with the incubated microcosms. The qPCR assays ( Fig. 3a ) of the archaeal 16S rRNA genes showed that (1) the original production water contained mostly the order Methanobacteriales and a smaller population of Methanosarcinales ; (2) the control microcosm was similarly dominated by hydrogenotrophic methanogens affiliated with the order Methanobacteriales ; whereas (3) the CO 2 -injected microcosms differed and were dominated by the order Methanosarcinales , many of which are acetoclastic methanogens. Clone library analyses supported the qPCR results. In the original production water and control microcosm, the genus Methanothermobacter dominated the archaeal community ( Fig. 3b and Supplementary Table S4 ). The control microcosm bacterial community was dominated by a limited number of phylotypes that includes the genus Thermacetogenium [17] , a known syntrophic acetate-oxidizing bacterium (99.8% sequence similarity) ( Supplementary Table S5 ). In contrast, all archaeal clones in the CO 2 -injected microcosms were affiliated with the acetoclastic species Methanosaeta thermophila strain PT (99% sequence similarity) ( Fig. 3b and Supplementary Table S4 ). In addition, in the CO 2 -injected microcosms, heterotrophic fermentative bacteria such as Coprothermobacter proteolyticus dominated in the bacterial community and the known syntrophic acetate-oxidizing bacteria disappeared ( Supplementary Table S5 ). These results clearly demonstrated that the main constituents of the control microcosm methanogenic microbial community were hydrogenotrophic methanogens and syntrophic acetate-oxidizers; CO 2 injection changed the community and led to the dominance of acetoclastic methanogens. These findings are consistent with the change in methanogenic pathways assessed by the stable isotope tracer experiment. 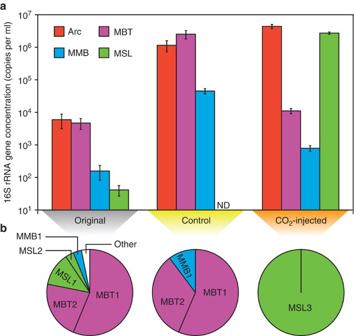Figure 3: Archaeal methanogenic community compositions. Archaeal methanogenic community compositions in the original production water, control (day 116) and CO2-injected microcosms (day 103). (a) The 16S rRNA gene copy concentrations of the domainArchaea(Arc), the ordersMethanobacteriales(MBT),Methanomicrobiales(MMB), andMethanosarcinales(MSL) quantified by qPCR assays. ND, not detected. (b) Relative abundance of archaeal clones. MBT1:Methanothermobacter thermautotrophicusKZ3-1 (DQ657903) (>99% similarity), MBT2:Methanothermobacter wolfeiiKZ24a (DQ657904) (>95% similarity), MSL1:Methanosaetasp. (AJ133791) (99% similarity), MSL2:Methanolobus psychrophilusR15 (EF202842) (98% similarity), MSL3:Methanosaeta thermophilaPT (AB071701) (99% similarity), MMB1:Methanoculleus receptaculiZC-3 (DQ787475) (99% similarity), Other:Thermococcus litoralisDSM5474 (AY099180) (99% similarity). Details of archaeal clone library analysis are shown inSupplementary Table S4. Figure 3: Archaeal methanogenic community compositions. Archaeal methanogenic community compositions in the original production water, control (day 116) and CO 2 -injected microcosms (day 103). ( a ) The 16S rRNA gene copy concentrations of the domain Archaea (Arc), the orders Methanobacteriales (MBT), Methanomicrobiales (MMB), and Methanosarcinales (MSL) quantified by qPCR assays. ND, not detected. ( b ) Relative abundance of archaeal clones. MBT1: Methanothermobacter thermautotrophicus KZ3-1 (DQ657903) (>99% similarity), MBT2: Methanothermobacter wolfeii KZ24a (DQ657904) (>95% similarity), MSL1: Methanosaeta sp. (AJ133791) (99% similarity), MSL2: Methanolobus psychrophilus R15 (EF202842) (98% similarity), MSL3: Methanosaeta thermophila PT (AB071701) (99% similarity), MMB1: Methanoculleus receptaculi ZC-3 (DQ787475) (99% similarity), Other: Thermococcus litoralis DSM5474 (AY099180) (99% similarity). Details of archaeal clone library analysis are shown in Supplementary Table S4 . Full size image Thermodynamic constraints on methanogenic reactions To elucidate the underpinning mechanisms of the shift in methanogenic pathways in conjunction with microbial community transition by injecting CO 2 , we conducted thermodynamic calculations for the following reactions under various partial pressures of CO 2 : acetate oxidation, hydrogenotrophic methanogenesis and acetoclastic methanogenesis. The thermodynamics showed that hydrogenotrophic methanogenesis becomes energetically more favorable with increasing CO 2 partial pressure, whereas acetate oxidation and acetoclastic methanogenesis become less favorable ( Fig. 4a ). However, acetoclastic methanogenesis is less sensitive to high CO 2 partial pressure than acetate oxidation because acetate oxidation produces two moles of CO 2 per mole of acetate, whereas acetoclastic methanogenesis produces one mole of CO 2 . The ΔG values calculated for the three reactions in the control and CO 2 -injected microcosms showed that acetate oxidation in the CO 2 -injected microcosm would be endergonic ( Fig. 4a and Table 1 ), indicating that syntrophic acetate oxidation coupled with hydrogenotrophic methanogenesis could not proceed under high CO 2 partial pressures but acetoclastic methanogenesis could proceed. A cultivation experiment verified the effect of CO 2 partial pressure on microbes; a pure syntrophic defined coculture [17] of Thermacetogenium phaeum strain PB and Methanothermobacter thermoautotrophicus strain TM was also inhibited by increasing CO 2 partial pressure ( Supplementary Note 2 and Supplementary Fig. S4 ). 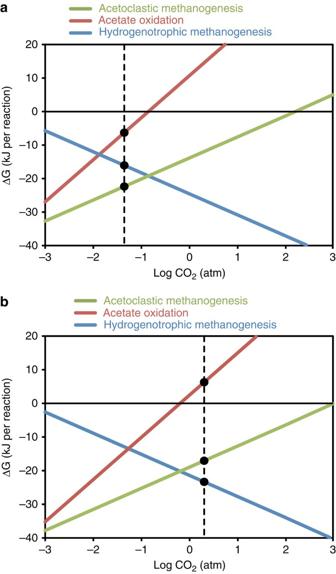Figure 4: CO2partial pressure effect on change in Gibbs free energy for acetate oxidation and methanogeneses. Effect of CO2partial pressure on the change in Gibbs free energy for acetate oxidation, hydrogenotrophic methanogenesis and acetoclastic methanogenesis. (a) The setup conditions are at 116 days of incubation in the control microcosm: acetate at 0.3 mM, methane at 0.51 atm, hydrogen at 1.5 × 10−4atm, pH=8.1, at 55 °C and 50 atm. (b) The setup conditions are at 77 days of incubation in the CO2-injected microcosm: acetate at 0.4 mM, methane at 0.66 atm, hydrogen at 1.2 × 10−4atm, pH=7.3, at 55 °C and 50 atm. Dashed lines indicate actual CO2partial pressures (0.04 and 2.0 atm) in the control and CO2-injected microcosms, respectively. Figure 4: CO 2 partial pressure effect on change in Gibbs free energy for acetate oxidation and methanogeneses. Effect of CO 2 partial pressure on the change in Gibbs free energy for acetate oxidation, hydrogenotrophic methanogenesis and acetoclastic methanogenesis. ( a ) The setup conditions are at 116 days of incubation in the control microcosm: acetate at 0.3 mM, methane at 0.51 atm, hydrogen at 1.5 × 10 −4 atm, pH=8.1, at 55 °C and 50 atm. ( b ) The setup conditions are at 77 days of incubation in the CO 2 -injected microcosm: acetate at 0.4 mM, methane at 0.66 atm, hydrogen at 1.2 × 10 −4 atm, pH=7.3, at 55 °C and 50 atm. Dashed lines indicate actual CO 2 partial pressures (0.04 and 2.0 atm) in the control and CO 2 -injected microcosms, respectively. Full size image Table 1 Thermodynamic parameters and Gibbs free energies of three reactions in the control and CO 2 -injected microcosms. Full size table This study illustrates the possibility that an increase in CO 2 partial pressure will change the microbial ecosystem in a deep subsurface high-temperature oil reservoir. Our results suggest that CO 2 injection into deep subsurface oil reservoirs can alter the in situ methanogenic pathway and lead to the dominance of acetoclastic methanogenesis. Acetate is often the most abundant organic acid in oil reservoirs [18] , [19] and an important intermediate in methanogenesis from crude oil [20] . Given that acetoclastic methanogenesis generally leads to a faster methanogenic reaction than syntrophic acetate oxidation coupled to hydrogenotrophic methanogenesis ( Supplementary Note 2 and Supplementary Fig. S4 ), the shift to this pathway may result in an acceleration of methane production in oil reservoirs as observed in this study ( Fig. 1a ). Furthermore, the thermodynamics, in theory, suggests that the shift to acetoclastic methanogenesis can ease the thermodynamic constraint of crude oil biodegradation ( Supplementary Fig. S5 ). Perhaps, the largest window of opportunity for crude oil biodegradation via acetoclastic methanogenesis alone [21] may lend further support to the hypothesis that CCS may increase energy recovery in the form of methane through crude oil biodegradation. Our results present a possibility of CCS for enhanced microbial energy production in deep subsurface environments that can mitigate global warming and energy depletion at the same time. To date, very little is known about the influence of CO 2 sequestration on the subsurface microbial communities and their functions, despite their important contribution to global biogeochemical processes [22] , [23] . This study would intrigue not only geochemists but also microbiologists for further investigation of CCS in connection with utilization of microbial activities in deep subsurface. Study site and sampling Yabase oil field is one of the oldest and largest onshore oil fields in Japan, located in Akita Prefecture (39° 42′N, 140° 5′E). Currently, the oil field is almost depleted and characterized by high overall water cut (~90% basic sediment and water). The main reservoir rocks are tuffaceous sandstone of Miocene–Pliocene age. The depth of the oil horizon ranges from 1000 to 1300, m, with in situ temperature and pressure estimated to be 53–65 °C and 5 MPa, respectively. In Yabase oil field, there are some production wells in which crude oil along with production water has been produced by pumping. In this study, reservoir samples were collected from one of the wells where water injection to enhance oil recovery has never been applied. The samples were taken from production flow at the wellhead by discharging the fluid mixture through a metal tube into gas-tight glass bottles flushed in advance with nitrogen gas in September 2009. Immediately before each bottle was sealed, the headspace was flushed and pressurized with nitrogen gas to minimize air contamination. The samples were maintained at 50°C for 3 days until use. Geochemical characteristics of the production water and gas sample from this reservoir have been previously described in the study by Mayumi et al. [15] Briefly, the water had low salinity (Cl − ; 4690, mg l −1 ) and −239 mV of reduction potential, and concentrations of nitrate and sulfate as electron acceptors were 14.5 μM and below 0.5 mM, respectively. Gas compositions of the sample collected from the production flow were H 2 : 0.1%, CO 2 : 2.4%, CH 4 : 77.2%, C 2 H 6 : 10.8%, C 3 H 8 : 5.2%, i- C 4 H 10 : 0.8% and n- C 4 H 10 : 1.5%. Microcosms Six microcosms were prepared with 800 ml of production water and 8 ml of crude oil in 1 l sterile stainless-steel cylinder bottles (304L-HDF4-1000; Swagelok, Ohio, USA) and stable isotope tracers were added as described in Supplementary Fig. S1 . Control microcosms were pressurized with nitrogen gas, and CO 2 -injected microcosms were pressurized with N 2 /CO 2 (90:10; δ CO2 =−34.8‰) at 5 MPa. Before pressurization of CO 2 -injected microcosms, sodium bicarbonate (δ NaHCO3 =−4.2‰) was added to a final concentration of 74 mM to mimic in situ conditions where formation water is highly buffered due to the presence of minerals such as calcite (CaCO 3 ) and dolomite (CaMg(CO 3 ) 2 ) in oil reservoirs [9] , [12] . The microcosms were incubated at 55 °C, and the mixing ratios of CH 4 and CO 2 in the headspace gases and organic acids in production water were periodically measured with a gas chromatograph and an ion chromatograph [15] . H 2 concentrations in the headspace gases were measured with an EAGanalyzer gas chromatograph equipped with a semiconductor detector (Sensortec Co., Ltd., Shiga, Japan). Carbon isotope analysis Headspace gas and the incubated water were collected into gas-tight glass cylinder bottles and vials, respectively, from all microcosms periodically. Carbon isotopic compositions of CH 4 in gas-tight glass cylinder bottles were determined with a Finnigan gas chromatograph combustion isotope ratio mass spectrometer (GC-C-IRMS) consisting of a Hewlett Packard 5890 GC, a Finnigan MAT 252 IRMS and a ThermoQuest combustion interface (Thermo Finnigan Inc., Texas, USA). Carbon isotopic composition of DIC in the incubated water was measured after the addition of 1 M H 2 SO 4 to liberate total CO 2 . All measurements were conducted in triplicate, and the s.e. values were less than 1‰. The isotopic values were expressed in δ notation relative to the Vienna Pee Dee Belemnite (VPDB) standard. The values of isotopic fractionation ( ε C ) between DIC and CH 4 were determined by ε C =(δ CH4 −δ DIC )/(1+δ DIC /10 3 ). Molecular biological analyses Molecular analyses were carried out for the original production water and incubated water from [2- 13 C]-acetate labeled microcosms (at day 116 and 103 for the control and the CO 2 -injected microcosms, respectively). Total DNA was extracted from a 0.22-μm-pore-size polycarbonate membrane filter (Millipore, MA, USA), concentrating 250 ml of the original production water, 15 ml of the control microcosm water and 40 ml of the CO 2 -injected microcosm water, using a FastDNA Spin kit (MP Biomedicals, CA, USA) according to the manufacturer’s protocol. Bacterial and archaeal 16S rRNA genes were amplified with primer sets Eub8F/Univ1490R [24] and Ar109F [25] /Univ1490R, respectively. PCR products were cloned using the pT7 Blue T-vector kit (Novagen, CA, USA). Clones were randomly selected (in archaeal libraries, original production water; 32 clones, control microcosm; 39 clones, CO 2 -injected microcosm; 35 clones, in bacterial libraries, original production water; 49 clones, control microcosm; 92 clones, CO 2 -injected microcosm; 84 clones), and the inserted 16S rRNA gene was directly amplified with T7 promoter primer and U-19mer primer (Novagen). Sequence analysis of 16S rRNA genes was carried out with a BigDye Version 3.1 reaction on an ABI3730xl DNA Analyzer (Applied Biosystems, CA, USA). Chimeric sequences were detected with the Bellerophon server [26] and removed from the sequence data sets. To group the OTUs and draw rarefaction curves, sequences were analyzed using FastGroupII program [27] with 97% sequence similarity. Representative sequences from each OTU were compared with those in public databases using the Seqmatch program from the Ribosomal Database Project (Release 10, Update 12) to identify the nearest neighbors. The specific primer and probe set for archaea, hydrogenotrophic methanogens (the orders Methanobacteriales and Methanomicrobiales ), and acetoclastic methanogens (the order Methanosarcinales ) used in quantitative real-time PCR to determine the 16S rRNA gene copy numbers were previously designed in the study by Yu et al. [28] All real-time PCR assays were performed with iCycler iQ using the iQ Supermix reaction kit (Bio-Rad, California, USA), as previously described in the study by Mayumi et al. [15] Standard curves for each assay were constructed using nearly full-length 16S rRNA gene fragments amplified from Methanothermobacter thermautotrophicus strain delta H (DSM 1053) for the Archaea and the Methanobacteriales assays, Methanoculleus bourgensis strain MS2 (DSM3045) for the Methanomicrobiales assay, Methanosaeta thermophila strain PT (DSM 6194) for the Methanosarcinales assay. Thermodynamics calculations Gibbs free energy calculations were made according to the study by Dolfing et al. [21] Temperature corrections were made with the Gibbs–Helmholz equation according to ΔG o Tact =ΔG o Tref . ( T act / T ref )+ΔH o Tref ·( T ref − T act )/ T ref with T in K; T act =328.15 K, T ref =298.15 K. The effect of pressure on ΔG (in kJ per reaction) was approximated as ΔG o Tref,Pact =ΔG o Tref,Pref +ΔV o ·(P act −P ref )/10000 where ΔG o Tref,Pact is the Gibbs free energy of reaction at the reference temperature (298.15 K) and in situ pressure (5 MPa; 50 atm), ΔG o Tref,Pref is the standard Gibbs free energy of reaction at the reference temperature and pressure (0.1 MPa; 1 atm), P act is the in situ pressure in atm, P ref is the reference pressure in atm and ΔV o is the partial molar volume change of the reaction at the reference temperature and pressure in cm 3 mol −1 , as outlined in the study by Wang et al. [29] . The calculations were made for acetate (p K a=4.75) at the appropriate pH values [30] . For the reaction CO 2 +4H 2 →CH 4 +2H 2 O, ΔV o =−62.3; for CH 3 COO − +H + +2H 2 O→4H 2 +2CO 2 , ΔV o =92.25; for CH 3 COO − +H + →CH 4 +CO 2 , ΔV o =29.95. Neglecting activity coefficients yields an error in calculated Gibbs free energy values of at most 2 kJ mol −1 for all reported values at an ionic strength of 0.1 M (Debye–Huckel calculations). Accession codes: All 16S rRNA gene sequences obtained in this study have been deposited at DDBJ under accession numbers AB668482 – AB668513 and AB710350 – AB710376 . How to cite this article: Mayumi, D. et al. Carbon dioxide concentration dictates alternative methanogenic pathways in oil reservoirs. Nat. Commun. 4:1998 doi: 10.1038/ncomms2998 (2013).